RETRACTED ARTICLE: Production of viable chicken by allogeneic transplantation of primordial germ cells induced from somatic cells The allogeneic transplantation of primordial germ cells (PGCs) derived from somatic cells overcomes the limitation of avian cloning. Here, we transdifferentiate chicken embryo fibroblasts (CEFs) from black feathered Langshan chickens to PGCs and transplant them into White Plymouth Rock chicken embryos to produce viable offspring with characteristics inherited from the donor. We express Oct4 / Sox2 / Nanog / Lin28A ( OSNL ) to reprogram CEFs to induced pluripotent stem cells (iPSCs), which are further induced to differentiate into PGCs by BMP4/BMP8b/EGF. DNA demethylation, histone acetylation and glycolytic activation elevate the iPSC induction efficiency, while histone acetylation and glycolytic inhibition facilitate PGCs formation. The induced PGCs (iPGCs) are transplanted into the recipients, which are self-crossed to produce 189/509 somatic cells derived chicken with the donor’s characteristics. Microsatellite analysis and genome sequencing confirm the inheritance of genetic information from the donor. Thus, we demonstrate the feasibility of avian cloning from somatic cells. Asexual propagation with somatic cell cloning has been carried out in more than 20 kinds of mammals [1] , [2] . However, this technique has never been successfully applied in avian species due to their specific oviparous reproductive pattern, which prevents somatic cell nuclear transfer [3] . Technical limitations have blocked research progress in the field of avian genetics, developmental biology and embryonic manipulations for a long period of time [4] . Allogeneic transplantation of chicken primordial germ cells (PGCs) was shown to produce offspring [5] and may be used for cloning methods in avian species. The current method of PGC transplantation requires 5–10 × 10 3 PGCs for each recipient, but only 3–5 × 10 3 PGCs can be harvested from a 4.5-day-developed chick gonad, which is insufficient for the requirements [6] , [7] . Somatic cells are easily available in large quantities and proliferate rapidly in vitro. In a single chick embryo incubated for 9–11 days, 10 7 chicken embryo fibroblasts (CEFs) can be harvested [4] . Hence, transdifferentiation of CEFs to PGCs may overcome the limitation of insufficient PGCs from chicken embryos for avian cloning, which will help to maintain poultry germplasm resources and may even restore endangered species [8] , [9] . Moreover, CEFs are easily genetically modified [10] , which will help produce transgenic chickens and develop optimized poultry breeds. In general, the establishment of a strategy for reprogramming CEFs to PGCs will have potential industrial applications in the future. Several studies have attempted to induce PGCs from skin-derived stem cells (SDSCs) in mammals. In mice, PGCs were induced by B27, epidermal growth factor (EGF), and basic fibroblast growth factor (bFGF) with an efficiency of 7% [11] , which was increased to 61.9% by addition of fetuin, retinoic acid (RA), bone morphogenetic protein 4 (BMP4), and activin A [12] . In a porcine model, reprogrammed PGCs were induced by the addition of follicular fluid, insulin transferrin selenium (ITS) and follicle-stimulating hormone (FSH) [13] , [14] . In humans, fetuin, ITS, EGF, activin A, and BMP4 were reported to successfully induce PGC formation [15] , [16] . In addition, embryonic stem cells (ESCs) were induced to differentiate into PGCs when cocultured with BMP4-expressing trophoblasts in mice (2.9%) and finally became functional sperm. Studies have shown that addition of components such as BMP4, BMP8b or LIF could increase the PGC induction rate to 13.5%–30% [8] , [9] , [17] , with successful production of offspring in mice [18] , [19] . Compared with that of mammals, chicken PGC induction is rarely reported. Overexpression of Cvh in chicken ESCs could generate PGC-like cells, with an efficiency of only 0.5% [20] . Later studies on PGC induction with BMP4 and RA also had a low efficiency of >10% [21] . Most importantly, induction of PGCs from somatic cells and the production of cloned offspring have never been achieved in chickens. In previous studies, we described the successful induction of chicken ESCs into PGCs with BMP4 in vitro [22] . However, ESCs are also difficult to isolate and cannot be easily transformed into PGCs [23] . Lu et al. demonstrated that CEFs can be induced to induced pluripotent stem cells (iPSCs) with human POU5F1, NANOG, SOX2, LIN28, KLF4 , and C-MYC genes [24] , and these cells expressed several PGC marker genes. However, no offspring were reported to be produced after in vivo transplantation. Hence, the development of an effective approach for PGC induction in vitro is urgently needed to address the limitations in avian cloning. This study aims to effectively produce viable chickens with donor’s characteristics by transplantation of iPGCs derived from somatic cells. Here, we reprogram CEFs from black feathered Langshan chickens to iPSCs and induce them to develop into iPGCs, which are transplanted into White Plymouth Rock chicken embryos to produce functional sperm or oocytes. With self-crossing, the recipients produce offspring, which are confirmed to inherit genetic information from the donor. This study reports the production of offspring from avian somatic cells, which overcomes the threshold in genetically uniform individual replication in avian species. CEFs can be reprogrammed to iPSCs We isolated CEFs from black feathered Langshan chickens and transfected them with Oct4/Sox2/Nanog/Lin28A ( OSNL ) (Fig. 1a and Supplementary Fig. 1A, B ). Morphological changes and pluripotent gene expression were monitored for 21 consecutive days (Fig. 1b, c ). On day 5, the cells became round and began to cluster. On day 15, typical iPSC morphology appeared. On day 17, cell clones displayed clear boundaries and spherical shapes, similar to ESCs. Analysis of pluripotent gene expression showed that on day 3, exogenous OSNL expression reached its peak and initiated endogenous pluripotent gene expression (Supplementary Fig. 1C ). The expression of the endogenous Oct4 , Sox2 , and Nanog genes increased gradually to a peak on day 18. Lin28A expression fluctuated, with a peak appearing on days 10 and 21 (Fig. 1c ). SSEA-1-positive cells were observed on day 21 at a rate of 1.45% ± 0.30 (Supplementary Fig. 1D ). Fig. 1: CEFs can be reprogrammed to iPSCs using OSNL factors. a Schematic diagram of a 21-day iPSC reprogramming process in vitro. The different colored dots represent the four genes of OSNL, OSNL represent Oct4, Sox2 Nanog , and Lin28A . The yellow cells represent CEF, and the blue cells represent iPS. b Morphological characterizations of CEF reprogramming to iPSCs from days 1 to 19, D means day. Scale bar: 50 μm ( n = 3 independent experiments). c qRT-PCR evaluation of endogenous reprogramming gene expression from days 0 to 21. A schematic diagram of the primers designed for endogenous OSNL gene expression is shown in Supplementary Fig. 1A . CEFs were used as a negative control (data are shown as mean ± SEM, statistically analyzed by unpaired two-tailed t -test * p < 0.05, ** p < 0.01, *** p < 0.001, n = 3 independent experiments). Full size image As epigenetic changes have been reported to influence iPSC formation in mammals [25] , we then evaluated the DNA methylation and histone acetylation status of endogenous pluripotent genes during iPSC reprogramming. The results indicated gradual demethylation of the Oct4 , Sox2 , and Nanog promoters by 39.14%, 49.33%, and 27.14% from days 0 to 20, respectively. No major change in DNA methylation was observed in the Lin28A promoter region (Fig. 2a ). In contrast, the concentration of histone acetyltransferase (HAT) was increased from 25.43 ± 1.89 ng/mL on day 0 to its peak of 81.84 ± 5.47 ng/mL on day 15 (Fig. 2b ). Regarding the epigenetic changes observed, we added the DNA methylase inhibitor vitamin C (VC) and/or the histone deacetylase transferase inhibitor valproic acid (VPA) to the OSNL induction system. VC or VPA increased the number of iPSC clones, while VC/VPA synergistically increased the number of iPSC clones from 26 ± 2.56 to 69 ± 3.00 ( p < 0.01; Fig. 2c, d ), with the percentage of SSEA-1-positive cells increasing from 1.45 ± 0.30% to 13.00 ± 0.14% ( p < 0.01; Fig. 2e ). The HAT concentration, as well as the expression of the pluripotent marker genes Nanog , Oct4 , Sox2 , Klf , and Rps17 , was elevated in the obtained cells (Fig. 2f, g ). These data suggested that DNA hypomethylation and histone hyperacetylation contribute to iPSC formation. Fig. 2: Optimizing the CEF reprogramming system for chicken iPSC production. a DNA methylation status evaluated by bisulfite sequencing of the OSNL gene promoter regions during iPSC reprogramming from day 0 to day 21, D means day. ESCs were used as the control. Black dots represent methylated sites, and white dots represent unmethylated sites, and ‘×’ represents undetected sites ( n = 10 repeats). b ELISA evaluation of histone acetyltransferase (HAT) concentrations from day 0 to day 21 during iPSC formation, ( n = 3 independent experiments). c Number of iPSC clones counted after adding the DNA methylase inhibitor VC and/or the histone deacetylase transferase inhibitor VPA to the reprogramming medium on day 21, VC vitamin C, VPA valproic acid. (data are shown as mean ± SEM, n = 3 independent experiments, * p < 0.05, ** p < 0.01, *** p < 0.001, one-way ANOVA). d Morphological evaluation of iPSC clones on day 21, Scale bar: 60 μm, ( n = 3 independent experiments). e Percentage of SSEA-1-positive cells on reprogramming day 21, (data are shown as mean ± SEM, n = 3 independent experiments, ** p < 0.01, *** p < 0.001, one-way ANOVA). f Enzyme-Linked Immunosorbent Assay (ELISA) evaluation of HAT concentration to show the change in histone acetylation status after the addition of VC and/or VPA. CEFs were used as the controls, (data are shown as mean ± SEM, n = 3 independent experiments, ** p < 0.01, *** p < 0.001, one-way ANOVA). g qRT-PCR evaluation of the expression of the pluripotent marker genes Nanog , Oct4 , Sox2 , Klf4 , and Rps17 . (Data are shown as mean ± SEM, n = 3 independent experiments, * p < 0.05, ** p < 0.01, *** p < 0.001, one-way ANOVA). Full size image In addition to epigenetic modifications, energy supply was recently reported to improve somatic cell reprogramming [26] , indicating the involvement of glycometabolism in iPSC formation. To test this hypothesis, we added the glycolytic activator 2i (PD0325901and SB431542) or inhibitor VK3 (Vitamin K3) to the OSNL system. On day 21, more iPSC clones appeared in the 2i-treated group than in the control group ( p < 0.05; Fig. 3a ). The proportion of SSEA-1-positive cells increased to 11.62%, and lactic acid glycolytic products were observed to accumulate in these cells (Fig. 3b and Supplementary Fig. 2 ). Conversely, VK3 reduced the number of SSEA-1-positive cells by five times compared to that of the control group (Fig. 3b ). To further assess the relationship between glycolysis and cell pluripotency, we used ESCs and CEFs as the positive and negative controls, respectively. As a result, VK3 added to the ESC culture medium decreased the expression of the Oct4 , Sox2 , and Nanog genes (Fig. 3c ), whereas a glycolytic activator added to the CEF medium increased the expression of these genes (Fig. 3d ). These results demonstrated that glycolysis enhances iPSC formation by activating the expression of endogenous pluripotent genes. Fig. 3: Glycolytic activation facilitates chicken iPSC formation. a Morphological evaluation and statistical analysis of iPSC clones with glycolytic activation (2i: PD0325901and SB431542) or inhibition (VK3: vitamin K3) in OSNL -induced iPSC formation. Scale bar: 60 m. (Data are shown as mean ± SEM, n = 3 independent experiments, ** p < 0.01, *** p < 0.001, one-way ANOVA). b . Flow cytometric analysis of SSEA-1-positive cells in the induced cells with glycolytic activation or inhibition, (data are shown as mean ± SEM, n = 3 independent experiments, ** p < 0.01, *** p < 0.001, one-way ANOVA). c , d qRT-PCR evaluation of the expression of the pluripotent genes Oct4 , Sox2 , Nanog , and Lin28A in ESCs ( c ) and CEFs ( d ), (data are shown as mean ± SEM, n = 3 independent experiments, * p < 0.05, ** p < 0.01, *** p < 0.001, one-way ANOVA). Full size image iPSCs show ESC-like characteristics We performed RNA-seq to evaluate the similarities between the iPSCs and ESCs (Fig. 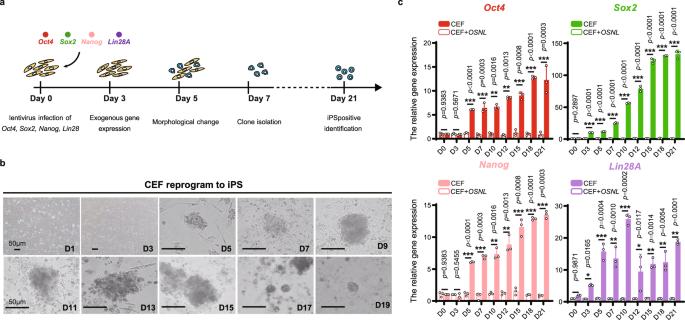Fig. 1: CEFs can be reprogrammed to iPSCs usingOSNLfactors. aSchematic diagram of a 21-day iPSC reprogramming process in vitro. The different colored dots represent the four genes ofOSNL, OSNLrepresentOct4, Sox2 Nanog, andLin28A. The yellow cells represent CEF, and the blue cells represent iPS.bMorphological characterizations of CEF reprogramming to iPSCs from days 1 to 19, D means day. Scale bar: 50 μm (n= 3 independent experiments).cqRT-PCR evaluation of endogenous reprogramming gene expression from days 0 to 21. A schematic diagram of the primers designed for endogenousOSNLgene expression is shown in Supplementary Fig.1A. CEFs were used as a negative control (data are shown as mean ± SEM, statistically analyzed by unpaired two-tailedt-test *p< 0.05, **p< 0.01, ***p< 0.001,n= 3 independent experiments). 4a and Supplementary Table 1 ). Unsupervised hierarchical clustering based on genes related to ESC development was applied. Principal component analysis (PCA) showed that the induced iPSCs had a more similar expression pattern to ESCs in the VC/VPA and 2i groups than in the OSNL group, which was further confirmed by correlation analysis (Fig. 4b, c ). Gene Ontology (GO) and Kyoto Encyclopedia of Genes and Genomes (KEGG) analysis indicated significant enrichment of the differentially expressed genes (DEGs) of iPSCs vs CEFs in the terms and signaling pathways related to stem cell development [27] , [28] , while no such enrichment was observed in the DEGs of iPSCs vs ESCs (Supplementary Fig. 3 ). Moreover, the expression pattern of the ESC marker genes in iPSCs was similar to that in ESCs but different from that in CEFs (Fig. 4d, e ). From the results above, we confirmed that the iPSCs induced by different induction systems all showed similar characteristics to ESCs. The cluster and correlation analysis, as well as the marker gene expression, indicated a close biological relationship of OSNL + VC/VPA-induced iPSCs to ESCs. We then used OSNL + VC/VPA for iPSC induction and obtained SSEA-1-positive cell lines showing chicken ESC-like characteristics (Supplementary Fig. 4 ). Fig. 4: iPSCs shows ESC-like biological characteristics. a Schematic diagram of RNA-seq analysis for iPSCs induced by OSNL , ONSL + 2i, and OSNL + VC/VPA. CEFs and ESCs were used as the negative and positive controls, respectively. Unsupervised hierarchical clustering based on ESC development-related genes was applied to analyze the similarities among the cell populations. Heatmap shows the expression profiles of the selected genes. Yellow cells represent CEF, red cells represent ESCs, green, blue, and purple cell represent iPSC from different induction system, and the dots with different colors represent independent samples from different groups for RNA-seq. The color key from blue to red indicates low to high gene expression. b , c Principal Component Analysis (PCA) ( b ) and correlation analysis ( c ) of iPSCs induced by OSNL , ONSL + 2i, and OSNL + VC/VPA to ESCs based on the genes selected in unsupervised hierarchical clustering. The color key from blue to white indicates short to long distances between samples. The colored dots represent sequencing data from individual cell samples. d , e Violin plot of ESC and CEF marker gene expression from the RNA-seq data of iPSCs from different groups, ESCs and CEFs. The solid lines at each end of the violin diagram represent the maximum and minimum values, respectively. The three dotted lines in the middle of the violin diagram represent the 75% percentile, the mean, and the 25% percentile in turn. Full size image Induction of iPSCs to iPGCs Based on the chicken ESC-PGC induction models established in our laboratory and others [22] , we first compared different compounds used for PGCs derived from ESCs. The results showed that the combination of BMP4, BMP8b, and EGF exhibited the highest induction rate of 26.20% ± 0.01 ( p < 0.01; Supplementary Fig. 5 ). In our previous work, de novo methylation was observed during ESC differentiation to PGCs in vivo [29] . Moreover, histone hyperacetylation and conversion of glycolysis to oxidative phosphorylation were reported to regulate the formation of iPGCs [26] . Here, we found that DNA demethylation reduced iPGC formation to 18.25% after addition of 5-aza-2′-deoxycytidine (5Aza-cd) to the medium, while VPA and VK3 increased iPGC formation to 29.70% and 34.90%, respectively, on day 4 (Supplementary Fig. 5G ). Thus, we concluded that DNA hypomethylation suppresses iPGC formation, while histone hyperacetylation and glycolytic inhibition facilitate this process, which could be used to optimize the iPGC induction system. To identify ESC-derived iPGCs, we performed RNA-seq (Supplementary Fig. 6A and Supplementary Table 1 ). Unsupervised hierarchical clustering based on genes related to PGC development showed that the BMP4-induced iPGCs had a different expression pattern than either ESCs or PGCs, whereas the BMP4/BMP8b/EGF-induced PGCs, as well as the cells with a combination with VPA, VK3, or 5Aza-cd, all showed high similarity to PGCs (Supplementary Fig. 6B ), which was further confirmed by correlation analysis (Supplementary Fig. 6C ). Moreover, PGC-related genes showed higher expression levels in iPGCs and PGCs than in ESCs. In addition, we further compared the marker genes of PGCs between different induction groups and observed that the BMP4/BMP8b/EGF-induced iPGCs showed a similar marker gene expression pattern to PGCs (Supplementary Fig. 6D ). The iPGCs obtained with BMP4/BMP8b/EGF exhibited better migration to the genital ridge following in vivo transplantation than the other cells (Supplementary Fig. 6E ). Hence, we concluded that BMP4/BMP8b/EGF-induced iPGCs are suitable for allogeneic transplantation. Based on the results above, we tried to induce iPSCs to iPGCs with BMP4/BMP8b/EGF. We selected clones of induced iPSCs on day 21 and established cell lines for each clone. The cell lines were prepared for later iPGC induction. We observed that the cells began to aggregate on day 2 and formed embryoid body-like structures on days 4–6. (Fig. 5a ). CVH expression and glycogen particles stained by periodic acid Schiff (PAS) were observed in the embryoid cells (Fig. 5b, c ). Flow cytometric analysis showed that the proportion of CVH-positive cells in the embryoid bodies increased from 4.6% ± 0.02 on day 2 to its highest level of 12.2% ± 0.01 on day 4 (Fig. 5d ) and was also affected by DNA methylation, histone acetylation, and glycolysis (Fig. 5e ). Quantitative real-time polymerase chain reaction (qRT-PCR) confirmed the increased expression of the PGC marker genes Cvh , Ckit , and Blimp1 , as well as the migration-related gene Cxcr4 ( p < 0.05; Supplementary Fig. 7 ). To further validate the results, we compared iPSC-derived iPGCs, ESC-derived iPGCs, PGCs, and ESCs with RNA-seq (Fig. 5f ). Unsupervised hierarchical clustering analysis showed that the iPGCs exhibited high similarity to PGCs in PCA and correlation analysis (Fig. 5g, h ). In addition, the iPSC-derived iPGCs showed a similar expression pattern of marker genes and migration to PGCs (Fig. 5i, j ). The results above indicated that the iPGCs induced from iPSCs are biologically similar to PGCs. Fig. 5: Induction of iPSCs to iPGCs. a Morphological evaluation of iPGCs induced from iPSCs with BMP4/BMP8b/EGF. ESCs were used as the control. Scale bar: 50 μm, ( n = 3 independent experiments). b iPSC-derived iPGCs stained with CVH as a PGC marker. PGCs were used as a positive control, and noninduced iPSCs were used as a negative control. Scale bar: 70 μm, ( n = 3 independent experiments). c Periodic acid-Schiff (PAS) staining of iPGCs, PGCs, and CEFs. The arrow shows the PAS positive iPGCs clones. Scale bar: 50 μm, ( n = 3 independent experiments). d Flow cytometric analysis of the CVH-positive iPGCs induced from iPSCs. The positive cells were counted on induction days 2, 4, 6, and 8, D means day. (data are shown as mean ± SEM, n = 3 independent experiments, *** p < 0.001, unpaired two-tailed t -test). e Flow cytometric evaluation of the iPGC formation rate in conditions with glycolytic activation, histone acetylation or DNA methylation, (data are shown as mean ± SEM, n = 3 indepe n dent experiments, ** p < 0.01, *** p < 0.001, unpaired two-tailed t -test). f Schematic diagram of RNA-seq analysis for iPGCs induced from iPSCs and ESCs. ESCs and PGCs were used as the controls. Unsupervised hierarchical clustering based on PGC development-related genes was applied to analyze the similarities among ESCs, ESC-derived iPGCs, iPSC-derived iPGCs, and PGCs. Heatmap shows the expression profiles of the selected genes. The color key from blue to red indicates low to high gene expression. White cells represent ESCs, red cells represent PGCs, blue cells represent iPS, cells with other colored represent iPGCs derived from different induction conditions. Dots with different colors represent independent samples from different groups for RNA-seq. g , h Principal Component Analysis (PCA) ( g ) and correlation analysis ( h ) of ESCs, ESC-derived iPGCs, iPSC-derived iPGCs, and PGCs based on the genes selected in unsupervised hierarchical clustering analysis. The color key from blue to white indicates short to long distances between samples. The colored dots represent sequencing data from individual cell samples. i Violin plot of PGC marker genes from RNA-seq data of ESCs, ESC-derived iPGCs, iPSC-derived PGCs and PGCs. The solid lines at each end of the violin diagram represent the maximum and minimum values, respectively. The three dotted lines in the middle of the violin diagram represent the 75% percentile, the mean, and the 25% percentile in turn. j ESCs, ESC-derived iPGCs, iPSC-derived iPGCs and PGCs were treated with pKH26 and injected into the recipients. The migration of the injected cells was evaluated by flow cytometric analysis of the pKH26-positive cells in isolated genital ridges. (Data are shown as mean ± SEM, n = 3 independent experiments, *** p < 0.001, one-way ANOVA). Full size image iPGCs can migrate to the genital ridge The derived iPGCs were purified by flow cytometry with the markers SSEA-1 and CVH. Then, the purified iPGCs, PGCs, ESCs, and CEFs were treated with pKH26 [30] and transplanted into chicken embryos on incubation day 2.5 (H&H 17). Real-time fluorescence of the genital ridge (day 4.5, H&H 26) revealed the appearance of red fluorescence (pKH26) in the iPGC and PGC groups (Fig. 6a and Supplementary Fig. 5D ). Similar fluorescence was also observed in the frozen sections of the genital ridges in the iPGC and PGC groups (Fig. 6b ). The green fluorescent protein (GFP) from the exogenous OSNL vectors was observed only in the iPGC group (Fig. 6a ), and this result was further confirmed by western blots (Supplementary Fig. 8 ). These findings demonstrated that the iPGCs induced from CEFs could migrate to chicken genital ridges after transplantation. Fig. 6: iPGCs migrate to the genital ridge after embryo transplantation. a Real-time fluorescence observation of genital ridges isolated from chicken embryos transplanted with iPGCs, PGCs, and CEFs. iPGCs, PGCs, and CEFs were treated with pKH26, showing red fluorescence before injection. Green fluorescence was expressed by the OSNL vectors carrying GFP originally transfected into CEFs. Scale bar: 2 mm. ( n = 9 chick embryos form three independent experiments). b Fluorescence observation of frozen embryonic genital ridge sections after iPGC, PGC, and CEF transplantation. Scale bar: 70 μm. ( n = 9 chick embryos form three independent experiments). Full size image Allogeneic transplantation of iPGCs and production of viable chickens The iPGCs derived from the CEFs of black feathered Langshan chickens were transplanted into 118 White Plymouth Rock chicken embryos (2.5 days). Forty-five chickens were obtained after hatching; these animals self-crossed and produced 189 somatic cell-derived offspring(positive) among 509 in total (positive rate 37.13%) (Fig. 7a, b ). These chickens were shown to be derived from the donor by the strain-specific microsatellite DNA markers LEI094, MCW004, and MCW104, with 11.48% homozygotes and 88.52% heterozygotes in the offspring (Supplementary Fig. 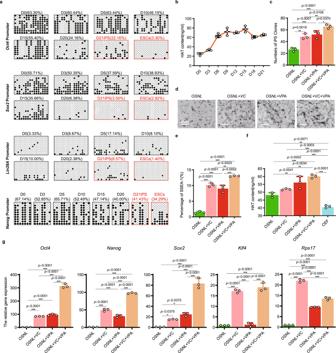Fig. 2: Optimizing the CEF reprogramming system for chicken iPSC production. aDNA methylation status evaluated by bisulfite sequencing of theOSNLgene promoter regions during iPSC reprogramming from day 0 to day 21, D means day. ESCs were used as the control. Black dots represent methylated sites, and white dots represent unmethylated sites, and ‘×’ represents undetected sites (n= 10 repeats).bELISA evaluation of histone acetyltransferase (HAT) concentrations from day 0 to day 21 during iPSC formation, (n= 3 independent experiments).cNumber of iPSC clones counted after adding the DNA methylase inhibitor VC and/or the histone deacetylase transferase inhibitor VPA to the reprogramming medium on day 21, VC vitamin C, VPA valproic acid. (data are shown as mean ± SEM,n= 3 independent experiments, *p< 0.05, **p< 0.01, ***p< 0.001, one-way ANOVA).dMorphological evaluation of iPSC clones on day 21, Scale bar: 60 μm, (n= 3 independent experiments).ePercentage of SSEA-1-positive cells on reprogramming day 21, (data are shown as mean ± SEM,n= 3 independent experiments, **p< 0.01, ***p< 0.001, one-way ANOVA).fEnzyme-Linked Immunosorbent Assay (ELISA) evaluation of HAT concentration to show the change in histone acetylation status after the addition of VC and/or VPA. CEFs were used as the controls, (data are shown as mean ± SEM,n= 3 independent experiments, **p< 0.01, ***p< 0.001, one-way ANOVA).gqRT-PCR evaluation of the expression of the pluripotent marker genesNanog,Oct4,Sox2,Klf4, andRps17. (Data are shown as mean ± SEM,n= 3 independent experiments, *p< 0.05, **p< 0.01, ***p< 0.001, one-way ANOVA). 9A and Supplementary Table 2 ). The weight of the donor-derived chickens was lower than that of their littermates, in accordance with the characteristics of these two breeds [31] (Fig. 7c ). The genetic relationship was further verified by whole-genome resequencing (Fig. 7d , Supplementary Fig. 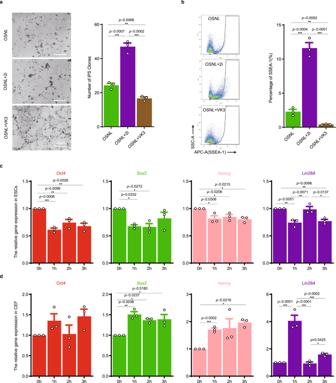Fig. 3: Glycolytic activation facilitates chicken iPSC formation. aMorphological evaluation and statistical analysis of iPSC clones with glycolytic activation (2i: PD0325901and SB431542) or inhibition (VK3: vitamin K3) inOSNL-induced iPSC formation. Scale bar: 60 m. (Data are shown as mean ± SEM,n= 3 independent experiments, **p< 0.01, ***p< 0.001, one-way ANOVA).b. Flow cytometric analysis of SSEA-1-positive cells in the induced cells with glycolytic activation or inhibition, (data are shown as mean ± SEM,n= 3 independent experiments, **p< 0.01, ***p< 0.001, one-way ANOVA).c,dqRT-PCR evaluation of the expression of the pluripotent genesOct4,Sox2,Nanog, andLin28Ain ESCs (c) and CEFs (d), (data are shown as mean ± SEM,n= 3 independent experiments, *p< 0.05, **p< 0.01, ***p< 0.001, one-way ANOVA). 9B, and Supplementary Table 3 ). Both phylogenetic tree and genetic similarity index (GSI) analyses showed that the positive offspring were closely related to both the donor and recipient strains (Fig. 7e, f ). 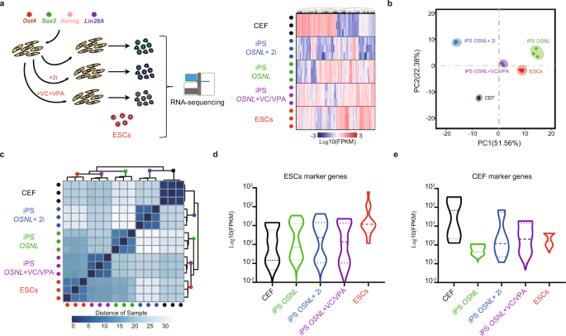Fig. 4: iPSCs shows ESC-like biological characteristics. aSchematic diagram of RNA-seq analysis for iPSCs induced byOSNL,ONSL+ 2i, andOSNL+ VC/VPA. CEFs and ESCs were used as the negative and positive controls, respectively. Unsupervised hierarchical clustering based on ESC development-related genes was applied to analyze the similarities among the cell populations. Heatmap shows the expression profiles of the selected genes. Yellow cells represent CEF, red cells represent ESCs, green, blue, and purple cell represent iPSC from different induction system, and the dots with different colors represent independent samples from different groups for RNA-seq. The color key from blue to red indicates low to high gene expression.b,cPrincipal Component Analysis (PCA) (b) and correlation analysis (c) of iPSCs induced byOSNL,ONSL+ 2i, andOSNL+ VC/VPA to ESCs based on the genes selected in unsupervised hierarchical clustering. The color key from blue to white indicates short to long distances between samples. The colored dots represent sequencing data from individual cell samples.d,eViolin plot of ESC and CEF marker gene expression from the RNA-seq data of iPSCs from different groups, ESCs and CEFs. The solid lines at each end of the violin diagram represent the maximum and minimum values, respectively. The three dotted lines in the middle of the violin diagram represent the 75% percentile, the mean, and the 25% percentile in turn. Moreover, the positive offspring contained specific single nucleotide polymorphisms (SNPs) from both the donor and recipient chickens (Supplementary Table 4 ). In addition, the copy number of the OSNL genes was higher in the positive offspring than in the donor and recipient chickens (Supplementary Fig. 9D ). EGFP expression was detected in the positive offspring (Supplementary Fig. 9E ). The results verified that the positive offspring were from transplanted iPGCs that were originally induced from CEFs donated by black feathered Langshan chickens. Fig. 7: Production and identification of somatic cell-derived chickens. a Schematic diagram of viable chicken production from somatic cells. Black feathered Langshan chickens are used as donors, White Plymouth Rock chicken are used as recipients. b i: Sexually mature White Plymouth Rock chickens that received iPGC transplantation in the embryo stage, as well as their positive ( n = 189) and negative offspring ( n = 320), showing black feathered, white feathered, black-white feathered, yellow feathered, and black-yellow feathered chickens; ii–x: offspring with similar appearance produced by the White Plymouth Rock chickens that received iPGC transplantation in the embryo stage. c Growth rate of the chickens positive for the clones compared with the negative chickens. (Data are shown as the mean ± SD, n = 5, 24, 22, 4 chicken in week 1, 2, 3, 4 in positive group, n = 1, 3, 12, 2 in week 1, 2, 3, 4 chicken in negative group, ** p < 0.01, unpaired two-tailed t -test). d Schematic diagram of whole-genome resequencing for the black feathered Langshan chicken, White Plymouth rock chicken and offspring. e Phylogenetic tree of donor black feathered Langshan chickens, recipient White Plymouth Rock chickens and offspring, Scale bar: 0.03 for genetic distance. Different colored dots represent individual sequenced samples. f Genetic similarity index (GSI) analysis of black feathered Langshan chickens, recipient White Plymouth rock chickens and offspring, the color key from blue to red indicates the similarities from low to high between samples. g Distribution of different single nucleotide polymorphism (SNP) loci in feather color-related genes in individuals with different feather color phenotypes. Horizontal axis represents for individuals. The vertical axis represents the proportion of variations. Scale bar represents the number of samples. Full size image In addition to the black feathered offspring, we also obtained chimeras of black-white feathered, yellow feathered and black-yellow feathered chickens (Fig. 7b ). Interestingly, many of them appeared similar to twins or multiples (Fig. 7b ). Based on these observations, we first sequenced the promoters and open reading frame (ORF) regions of two color-related genes, melanocortin 1 receptor ( MC1R ) [32] and tyrosinase ( TYR ) [33] . Base mutations in the promoter regions and exons of these two genes were detected in animals with all three feather color phenotypes (Supplementary Fig. 9F ). 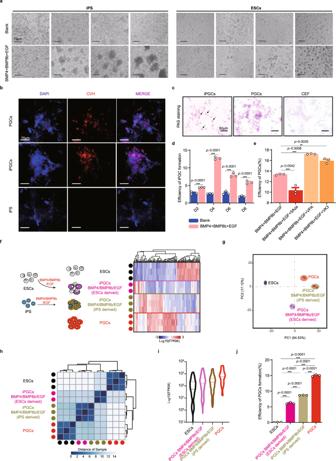Fig. 5: Induction of iPSCs to iPGCs. aMorphological evaluation of iPGCs induced from iPSCs with BMP4/BMP8b/EGF. ESCs were used as the control. Scale bar: 50 μm, (n= 3 independent experiments).biPSC-derived iPGCs stained with CVH as a PGC marker. PGCs were used as a positive control, and noninduced iPSCs were used as a negative control. Scale bar: 70 μm, (n= 3 independent experiments).cPeriodic acid-Schiff (PAS) staining of iPGCs, PGCs, and CEFs. The arrow shows the PAS positive iPGCs clones. Scale bar: 50 μm, (n= 3 independent experiments).dFlow cytometric analysis of the CVH-positive iPGCs induced from iPSCs. The positive cells were counted on induction days 2, 4, 6, and 8, D means day. (data are shown as mean ± SEM,n= 3 independent experiments, ***p< 0.001, unpaired two-tailedt-test).eFlow cytometric evaluation of the iPGC formation rate in conditions with glycolytic activation, histone acetylation or DNA methylation, (data are shown as mean ± SEM,n= 3 independent experiments, **p< 0.01, ***p< 0.001, unpaired two-tailedt-test).fSchematic diagram of RNA-seq analysis for iPGCs induced from iPSCs and ESCs. ESCs and PGCs were used as the controls. Unsupervised hierarchical clustering based on PGC development-related genes was applied to analyze the similarities among ESCs, ESC-derived iPGCs, iPSC-derived iPGCs, and PGCs. Heatmap shows the expression profiles of the selected genes. The color key from blue to red indicates low to high gene expression. White cells represent ESCs, red cells represent PGCs, blue cells represent iPS, cells with other colored represent iPGCs derived from different induction conditions. Dots with different colors represent independent samples from different groups for RNA-seq.g,hPrincipal Component Analysis (PCA) (g) and correlation analysis (h) of ESCs, ESC-derived iPGCs, iPSC-derived iPGCs, and PGCs based on the genes selected in unsupervised hierarchical clustering analysis. The color key from blue to white indicates short to long distances between samples. The colored dots represent sequencing data from individual cell samples.iViolin plot of PGC marker genes from RNA-seq data of ESCs, ESC-derived iPGCs, iPSC-derived PGCs and PGCs. The solid lines at each end of the violin diagram represent the maximum and minimum values, respectively. The three dotted lines in the middle of the violin diagram represent the 75% percentile, the mean, and the 25% percentile in turn.jESCs, ESC-derived iPGCs, iPSC-derived iPGCs and PGCs were treated with pKH26 and injected into the recipients. The migration of the injected cells was evaluated by flow cytometric analysis of the pKH26-positive cells in isolated genital ridges. (Data are shown as mean ± SEM,n= 3 independent experiments, ***p< 0.001, one-way ANOVA). Whole-genome resequencing analysis was further carried out, showing 674 phenotype-specific SNPs in black-white feathered chickens, 698 in yellow feathered chickens, and 966 in black-yellow feathered chickens (Supplementary Table 5 ), and similar SNPs appeared in the same phenotype (Supplementary Fig. 9C ). Furthermore, we screened specific SNPs in 15 feather color-related genes, and their unique combinations were observed in the three feather color phenotypes (Fig. 7h ). Based on these results, we confirmed that chickens with the same phenotype generated from CEFs belong to similar variant types. This phenomenon was not observed in the offspring generated by PGC transplantation (Supplementary Fig. 10 ). The results above demonstrated the production of viable chicken from iPGCs derived from CEFs. In this study, we produced viable chickens from somatic cells. Glycolytic inhibition and histone hyperacetylation were applied to optimize the induction system, which increased the number of iPGCs by 10 4 orders of magnitude. Microsatellite analysis and whole-genome resequencing fully confirmed that the somatic cell-derived chicken inherited genetic information from the donor. Our study demonstrates the possibility of chicken reproduction from somatic cells. The low iPSC induction efficiency is largely due to the poor reprogramming ability of CEFs. In addition to epigenetic modifications by DNA methylation and histone deacetylation, intracellular metabolism was shown to be involved in chicken iPSC formation [34] , [35] . In this study, suppression of intracellular glycolytic rate-limiting enzymes accelerated iPSC formation. This phenomenon is possibly due to GSK3-β inactivation and Nanog suppression by MAPK/ERK [36] , [37] , [38] , as well as suppression of GSK3-β activity by TGF-β phosphorylation [39] . Therefore, as the key kinase that promotes glycolysis, GSK3-β might promote iPSC formation by catalyzing glycolysis [40] . Previous studies have reported the application of BMP4/BMP8b/EGF to induce ESCs to iPGCs in mice [41] , which was also shown to be applicable in inducing iPSCs to iPGCs in our study. Moreover, we found that epigenetic regulation by addition of VC or VPA, as well as glycolytic inhibition with VK3, could significantly enhance PGC formation (from 12.2% to 16.41%). In addition, studies have shown that lncRNAs [42] , ubiquitination [43] , phosphorylation [44] , and histone methylation [45] promote iPGC formation, which should also be considered to optimize the iPGC induction system. In this study, we assessed the migration of iPGCs, PGCs, ESCs, and CEFs in vivo by pKH26. We only observed the red fluorescence of pKH26 in the genital ridges of the iPGC and PGC groups. Finally, somatic cell-derived chickens were produced as expected. The different feather color phenotypes might be due to the random insertion of exogenous OSNL lentivirus vectors, which disrupt the feather melanin diffusion gene E [46] , [47] . Evidence has also shown feather color-related gene mutations in different feather color phenotypes, which may also contribute to the characteristic segregation of feather color in offspring [32] , [33] . We found that 11.48% of the offspring were homozygotes with black feathers and should be generated by donor CEF-produced sperm and oocyte fertilization or the complementary effect of the insertion stie in melanin diffusion gene E, such as that found in the Benzer complementation test. The offspring were identified by breed-specific microsatellite DNA fingerprinting and whole-genome resequencing, which not only confirmed the inheritance of similar hereditary information from the donor chicken CEFs but also revealed the appearance of homozygotes. These results were consistent with self-crossing purification in Mendel’s law of separation. In general, the reason for character segregation of feather color in somatic cell-derived chickens is complicated, and the detailed molecular mechanisms require further study. In conclusion, we established an efficient system for CEF-iPSC-iPGC induction (Fig. 8 ). The obtained iPGCs could migrate and home to chicken genital ridges after transplantation, where they developed into functional sperm or oocytes to generate viable chickens. This method overcomes the technical limitations of avian somatic cell cloning and allows genetic modifications, large expansion of elite avian species and even restoration of endangered birds. Fig. 8: Schematic diagram of the viable offspring production derived from donor CEF. CEFs of black feathered Langshan chickens were induced to differentiate into iPGCs and injected into the embryos of White Plymouth Rock chickens. The injected iPGCs migrate to the genital ridge and develop into germ cells. The recipients with transplanted iPGCs produced viable offspring showing characteristics of black feathered Langshan chickens by self-crossing. Full size image Animal ethics statements Healthy black feathered Langshan chickens ( Gallus domestiaus ) and White Plymouth Rock chickens were selected for this study. All animals were housed in the Animal Facility of Yangzhou University. The use and care of animals complied with the guidelines of the Animal Advisory Committee at Yangzhou University. The ethics application was approved by the Ethics Committee of Yangzhou University. Cell isolation CEF was isolated from E9 chicken embryos (HH St. 35). After 9 days of incubation, the eggs were disinfected with Benzalkonium Bromide Solution (Nanchang Baiyun Pharmaceutical Co., Ltd., Nan Chang, China, H36021593) and 75% alcohol. The eggs were broken in a clean bench. The chicken embryos were taken out and washed two times with PBS to remove the head, limbs, internal organs and bones. The remaining tissue was shredded and digested repeatedly with 2 ml 0.25% trypsin (Gibco, New York, USA, 25200072) for 5 min, the digestion was terminated by 2 ml DMEM (Gibco, New York, USA, 10829018) containing 10% FBS (Gibco, New York, USA, 10099141), filtered with 400 mesh nylon cloth, the cell suspension was centrifuged for 6 min with 800× g , the supernatant was discarded, and the 3 ml DMEM (10%FBS) was added to re-suspend cells. In total, 1 × 10 6 cells/mL was spread in 60 mm cell petri dish and cultured at 37 °C in 5%CO 2 incubator. ESC was isolated from E0 chicken embryos (HH St. 1). The fertilized eggs were sterilized with Benzalkonium Bromide Solution and 75% alcohol, then the blastocyst was removed with a spoon and washed in PBS two times and filtered through 400 mesh, the suspension was centrifuged for 6 min with 800 × g , the supernatant was discarded, the cell precipitation was suspended with 3 ml ESC medium and transferred to the 60 mm cell petri dish at 37 °C, 5%CO 2 incubator for 24 h, then the supernatant was collected for subsequent culture. PGCs was isolated from E4.5 chicken embryos (HH St. 24). Eggs incubated for 4.5 days were sterilized with Benzalkonium Bromide Solution and 75% alcohol. The chicken embryos were taken in clean bench, and the genital ridge was taken under the microscope and shredded with scissors. The chopped tissues were collected and precipitated by centrifugation for 6 min with 800 × g . In all, 1 ml trypsin was used to digest the precipitation for 3 min, and then add the DMEM (10%FBS) to terminate the digestion. After filtration with 400 mesh nylon cloth, 800 × g centrifuged for 8 min, discarded the supernatant, precipitated, and re-suspended with 3 ml DMEM(10%FBS), then transferred to 60 mm cell culture dish at 37 °C, 5%CO 2 incubator for 40 min, the upper layer cells were taken for subsequent culture. Cell culture The isolated CEFs were cultured in DMEM (HyClone, Utah, USA, sh30243.01) containing 10% FBS (Gibco, New York, USA, 10099141). ESC medium contained 43.5 mL of Knockout-DMEM (Gibco, New York, USA, 10829018), 100 μL of gentamicin (Solarbio, Beijing, China, G8170), 0.2 μL of β-mercaptoethanol (Sigma, Missouri, USA, M3148), 200 μL of nonessential amino acids (Sigma, Missouri, USA, M7145), 1 mL of chicken serum (Gibco, New York, USA, 16110-082), 100 μL of SCF (Sigma, Missouri, USA, 300-07-10), 100 μL of bFGF (Sigma, Missouri, USA, F0291), 50 μL of LIF (Millipore, Massachusetts, USA, ESG1106), and 500 μL of penicillin (Solarbio, Beijing, China, P1400-100). ESC medium was removed after obvious cell clones appeared after iPSC induction (24-well plates). The cells were then washed with PBS 1–3 times, and 200 μL of Accutase (Gibco, New York, USA, 40506ES60) was added for a 5 min digestion. The cells were collected and centrifuged at 1000 × g for 8 min. Next, 1 mL of Accutase solution was added to the cell pellet for further digestion of the iPSC clones at 37 °C for 10 min. Then, the suspended cells were seeded into a new feeder layer for culture. A step-by-step protocol for CEF reprogramming, iPGC induction and offspring production from iPGCs via allotransplantation can be found at Nature Protocol Exchange [48] . CEF reprogramming to iPSCs A cDNA library of chicken ESCs was constructed according to the instructions of the HiScript® 1st Strand cDNA Synthesis Kit (Tiangen, Beijing, China, KR118). The CDSs of the OSNL genes were cloned into the pCDH-CMV-MCS-GFP vector (from our laboratory). The constructed vector was then subjected to double-enzyme digestion with EcoRI (NEB, Beijing, China, R3101) and BamHI (NEB, Beijing, China, R3136). The products were identified by 1% agarose (Tsingke, Beijing, China, TSJ001) gel electrophoresis and sequenced. After lentivirus encapsulation, 1.5 × 10 5 CEFs/well were seeded in a 24-well plate. When the cell density reached 60%, the OSNL four-factor lentiviral vector (1:1:1:1) was used to infect CEFs at a multiplicity of infection of 10 with 5 ng/mL polybrene (Santa Cruz, California, USA, SC-134220). After 24 h, the culture medium was replaced with DMEM containing 10% FBS and cultured for 72 h. The medium was then replaced by ESC medium. The cells were cultured until the 5th day and transferred to the CEF feeder layer treated with mitomycin C (MCE, New Jersey, USA, HY-13316). On the seventh day, cells were selected for single-cell clones under a stereomicroscope (Olympus, Tokyo, Japan, DP72). Single-cell clones were digested with Accutase for 10 min and then seeded on 96-well plates with feeder cells for amplification. The entire iPSC reprogram process lasted 21 days. iPSC Induction to iPGCs iPSC clones were picked by mouth pipetting on induction day 21. Then, the cell line for each clone was established and prepared for iPGC induction. The collected iPSCs were seeded in a 100-mm petri dish and adhered differentially for 45 min. The cell supernatant was harvested after removing the feeder cells in the iPSCs. iPSCs (5 × 10 4 cells/well) were seeded in a 24-well plate, and 40 ng/mL BMP4 (ProSpec, Rehovot, Israel, CYT-361), 40 ng/mL BMP8b (R&D, Minneapolis, USA, 9316-BP), and 50 ng/mL EGF (Thermo Scientific, Shanghai, China, PHG0314) were added. The medium was changed every other day, and changes in cell morphology were observed. The complete process lasted 6 days. The induced iPGCs were purified by flow cytometry with SSEA1 and CVH, which were then used for in vivo transplantation. RNA-seq Total RNA was isolated from iPSCs induced by different induction systems with ESCs as a positive control and CEFs as a negative control according to the manufacturer’s instructions (Supplementary Table 1 ). DNase I digestion was performed before purifying mRNA by enriching Oligo(dT) magnetic beads (Enriching Biotechnology, Ltd., Shanghai, China). The purified mRNA was sonicated, and first-strand cDNA was synthesized by six bp random primers. Second-strand cDNA was synthesized and purified. The sequencing library was constructed and sequenced by Illumina HiSeqTM 2500 and yielded 150-base paired-end reads. The read numbers of each sample were analyzed by eXpress software and normalized by estimating the size factors of the R package in DESeq (2012). The relative level of expression was normalized to fragments per kilobase of transcript per million mapped reads (FPKM) by Bowtie2. The p -value and log fold change were analyzed by the Nbinom test. After mapping the sequencing reads to the genome using HISAT2, the read counts of each gene were obtained by HTSeq-count. Then unsupervised hierarchical clustering was performed by euclidean distance through pheatmap package within gene read counts to analyze the similarity between different cell populations [49] , [50] , [51] . Briefly, all the DEGs were enriched in GO and KEGG items. The genes enriched in the items related to ESC (GO: 0072089, GO: 0019827 etc.) [52] , [53] , [54] or PGC (GO:0007281, GO:0008406 etc.) [17] , [55] development were collected and used for further analysis. The different expression patterns of all samples are displayed by a heatmap. During the analysis, the R packages ggplot2, Pca3d, and Pheatmap were used to draw box plots, PCA plots, and heatmaps, respectively. Whole-genome resequencing Blood samples were collected from parental black Langshan chickens and recessive white feathered chickens and offspring with different phenotypes (Supplementary Table 3 ). Sequencing and analysis were conducted by OE Biotech Co., Ltd. (Shanghai, China). The libraries were constructed with the TruSeq Nano DNA LT Sample Preparation Kit (Illumina, San Diego, CA, USA). Briefly, the genomic DNA was sonicated to obtain fragments with a length of ~350 bp using S220 focused ultrasonicators (Covaris, USA). Adapters were ligated onto the 3′ end of the sheared fragments. After PCR amplification and purification, the final libraries were sequenced on the Illumina HiSeq X Ten platform (Illumina, Inc., San Diego, CA, USA), and 150 bp paired-end reads were generated. The raw reads were subjected to a quality check and then filtered by fastp (Version 0.19.5) [56] . Clean reads were aligned to the reference genome (GCF_000002315.5) using Burrows-Wheeler Aligner (BWA, Version 0.7.12) [57] . During the analysis, GSI, evolutionary tree analysis and PCA were used to detect the genetic relationship between the offspring and black feathered Langshan chickens and White Plymouth Rock chickens. Quantitative real-time polymerase chain reaction Tissues and cells were homogenized in TRIzol Reagent, and total RNA was isolated according to the manufacturer’s instructions (Qiagen, Beijing, China, DP424). qRT-PCR was performed using a FastKing One-Step RT-PCR Kit with SYBR Green (Qiagen, Beijing, China, KR123), and the mRNA levels of related genes were measured by a CFX-Connect Real-time PCR detection system (Bio-Rad, California, USA, 7500fast). The expression levels were determined with a housekeeping gene ( β-actin ) using the 2 −ΔΔCt method. 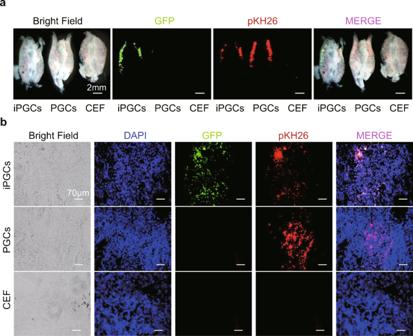Fig. 6: iPGCs migrate to the genital ridge after embryo transplantation. aReal-time fluorescence observation of genital ridges isolated from chicken embryos transplanted with iPGCs, PGCs, and CEFs. iPGCs, PGCs, and CEFs were treated with pKH26, showing red fluorescence before injection. Green fluorescence was expressed by theOSNLvectors carrying GFP originally transfected into CEFs. Scale bar: 2 mm. (n= 9 chick embryos form three independent experiments).bFluorescence observation of frozen embryonic genital ridge sections after iPGC, PGC, and CEF transplantation. Scale bar: 70 μm. (n= 9 chick embryos form three independent experiments). The qRT-PCR primers are listed in Supplementary Table 6 . Bisulfite sequencing analysis of DNA methylation Cell samples taken on days 0, 3, 5, 10, 15, 20, and 21 during iPSC induction, ESCs and iPSCs were collected separately for DNA extraction. Bisulfite conversion was carried out on 1 μg of isolated DNA from each sample using a DNA methylation kit (Tiangen, Beijing, China, DP215) according to the manufacturer’s instructions. The bisulfite-converted DNA was amplified by PCR with the primers listed in Supplementary Table 6 . PCR products were then purified using 1.5% agarose gel electrophoresis. The purified product was ligated with the pClone007 blunt simple vector according to the procedure of the pClone007 Blunt Simple Vector Kit (Qingke, Beijing, China, TSV-007S) and transformed into competent cells and coating plates. Ten clones were selected from each transformation plate for sequencing, and the sequencing results were compared online at http://quma.cdb.riken.jp/top/index.html (Beijing Qingke Xinye Biotechnology Co., Ltd., China). The changes in DNA methylation in the promoter regions of the Oct4, Sox2, Nanog , and Lin28A genes during iPSC formation were analyzed. ESCs and CEFs were utilized as controls. Flow cytometric analysis Cells harvested from different induction days were blocked with blocking buffer (PBS containing 10% fetal bovine serum; Gibco, New York, USA, 10270-106) for 2 h at 37 °C. The samples were incubated with antibodies against cell surface epitopes (SSEA1, R&D, Minneapolis, USA, IC2155T, 1:100–1000; MVH, Abcam, Cambridge, UK, ab13840, 1:100; CKIT, Thermo Fisher Scientific, Shanghai, China, 14-1172-81, 1:100) at 4 °C overnight, washed with PBS containing 0.1% Tween-20 (Solarbio, Beijing, China, T8220) three times, and then incubated with a fluorescence-coupled secondary antibody (goat anti-rabbit IgG FITC conjugated, CWBIO, Shanghai, China, CW0114S, 1:100; goat anti-mouse IgG H&L [TRICT], Abcam, Cambridge, UK, ab6786, 1:100) at 37 °C for 2 h. Then, the cells were washed with PBS containing 0.1% Tween-20 three times. 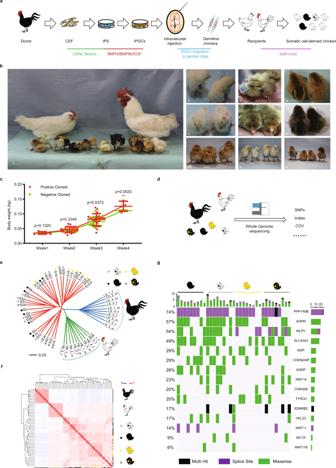Fig. 7: Production and identification of somatic cell-derived chickens. aSchematic diagram of viable chicken production from somatic cells. Black feathered Langshan chickens are used as donors, White Plymouth Rock chicken are used as recipients.bi: Sexually mature White Plymouth Rock chickens that received iPGC transplantation in the embryo stage, as well as their positive (n= 189) and negative offspring (n= 320), showing black feathered, white feathered, black-white feathered, yellow feathered, and black-yellow feathered chickens; ii–x: offspring with similar appearance produced by the White Plymouth Rock chickens that received iPGC transplantation in the embryo stage.cGrowth rate of the chickens positive for the clones compared with the negative chickens. (Data are shown as the mean ± SD,n= 5, 24, 22, 4 chicken in week 1, 2, 3, 4 in positive group,n= 1, 3, 12, 2 in week 1, 2, 3, 4 chicken in negative group, **p< 0.01, unpaired two-tailedt-test).dSchematic diagram of whole-genome resequencing for the black feathered Langshan chicken, White Plymouth rock chicken and offspring.ePhylogenetic tree of donor black feathered Langshan chickens, recipient White Plymouth Rock chickens and offspring, Scale bar: 0.03 for genetic distance. Different colored dots represent individual sequenced samples.fGenetic similarity index (GSI) analysis of black feathered Langshan chickens, recipient White Plymouth rock chickens and offspring, the color key from blue to red indicates the similarities from low to high between samples.gDistribution of different single nucleotide polymorphism (SNP) loci in feather color-related genes in individuals with different feather color phenotypes. Horizontal axis represents for individuals. The vertical axis represents the proportion of variations. Scale bar represents the number of samples. 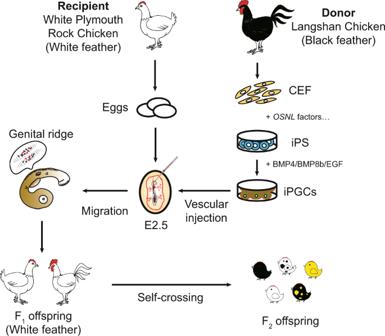Fig. 8: Schematic diagram of the viable offspring production derived from donor CEF. CEFs of black feathered Langshan chickens were induced to differentiate into iPGCs and injected into the embryos of White Plymouth Rock chickens. The injected iPGCs migrate to the genital ridge and develop into germ cells. The recipients with transplanted iPGCs produced viable offspring showing characteristics of black feathered Langshan chickens by self-crossing. The staining signal was analyzed by FACS LSRFortessa (BD Biosciences, USA) with a minimum of 10 4 events in each experiment. Alkaline phosphatase staining Alkaline phosphatase staining was performed using the Solarbio Alkaline Phosphatase kit (Solarbio, Beijing, China, G1480). After PBS washes, the iPSCs were treated with ALP fixed solution for 3 min and washed with ALP incubation solution for 15–20 min. Nuclei were stained with 1 mg/mL Hoechst 33342 (Invitrogen, California, USA, R37165) for 3–5 min after the cells were washed with PBS. Images were obtained using a fluorescence inverted microscope (Olympus, Japan, Tokyo, IX51). Cloning and analysis of short tandem repeats (microsatellites) Blood was collected from Langshan chickens (recessive white chickens) and offspring produced by allogeneic transplantation. DNA was isolated according to the procedure of the DNA extraction kit (Tiangen, Beijing, China, DP304). A 5-terminal FAM fluorescently modified primer (Supplementary Table 6 ) was synthesized based on the LEI094, MCW004, and MCW104 microsatellite loci. Preliminary quantification was determined by 1.5% agarose gel electrophoresis after PCR amplification and the internal standard liz500 to perform 3730xl capillary electrophoresis. GeneMapper software was used to analyze the capillary electrophoresis results. The PCR amplification system included 1 μL of DNA, 1 μL of Primer F, 1 μL of Primer R, 15 μL of master mix, and 12 μL of ddH 2 O. PCR amplification was performed with an initial denaturation of 94 °C for 2 min, followed by 35 cycles of denaturation at 94 °C for 10 s, annealing at 55 °C for 10 s and elongation at 72 °C for 10 s, ending with a final extension at 72 °C for 5 min (Beijing Qingke Xinye Biotechnology Co., Ltd., China). Enzyme-linked immunosorbent assay During the process of iPSC induction, cells were collected on days 0, 3, 6, 9, 12, 15, 18, and 21. During iPGC generation, cells were harvested on days 2, 4, 6, and 8. The collected cells were diluted to 1 × 10 6 cells/mL with PBS. A cell disruption system (ATPIO, Nanjing, China, ATPIO-1000D) was used to lyse the cells. The lysed cells were assessed at 450 nm to measure the HAT concentration using a chicken HAT ELISA kit (YL, Shanghai, China, GR-E63027). Western blot A total of 1 × 10 6 cells were treated with 200 μL of RIPA lysis buffer (CWBIO, Beijing, China, CW2333S) and 2 μL of protease inhibitor PMSF (Solarbio, Shanghai, China, P0100). Total protein was quantified using the Pierce BCA Protein Assay Kit (CWBIO, Beijing, China, CW0014S) and denatured at 100 °C for 10 min. Equal amounts of the lysates were fractionated by 12% SDS-PAGE (GenScript, Nanjing, China, M01210C). Proteins were transferred onto PVDF membranes (Solarbio, Shanghai, China, YA1701) using a Semi-Dry Electrophoretic Transfer Cell (Bio-Rad, California, USA, Trans-Blot ® SD). After the membranes were blocked overnight with 5% skim milk (Bio-Rad, California, USA, 1706404) and washed with TBST three times, they were probed with antibodies against GFP (CWBIO, Beijing, China, CW0087M, 1:1000) and β-actin (CWBIO, Beijing, China, CW0096M, 1:500). Goat anti-rabbit antibody (CWBIO, Beijing, China, CW0107S, 1:1000) and goat anti-mouse antibody (CWBIO, Beijing, China, CW0102S, 1:2000) were used as secondary antibodies. Uncropped blots can be found in the Source data file. Lactate production assay The lactic acid assay kit (Jiancheng Bioengineering Institute, Nanjing, China, A019-2-1) was used to determine lactate generation. The culture media supernatant was collected for lactate detection according to the manufacturer’s instructions. The absorbance was measured by a microplate spectrophotometer (Tecan, Switzerland, Infinite M200 Pro). The amount of lactate generated was calculated as follows: lactate generation (mM) = 3 (OD sample − OD blank )/(OD standard − OD blank ). Immunofluorescence staining Cells were fixed with 4% paraformaldehyde for 30 min at room temperature and permeabilized with 0.5% Triton X-100 (Solarbio, Beijing, China vT8200) for 10 min. The samples were then blocked with blocking buffer (PBS containing 10% fetal calf serum [FBS]) (Gibco, New York, USA, 10099141) at 37 °C for 2 h or 4 °C overnight. Primary antibodies diluted in blocking buffer were used for the samples and incubated at 37 °C for 2 h or 4 °C overnight. The samples were washed three times with PBS containing 0.1% Tween 20 (Solarbio, Beijing, China, T8220) followed by incubation with fluorescence-conjugated secondary antibodies diluted in blocking buffer for 2 h at 37 °C. The samples were washed three times with PBS containing 0.1% Tween 20. Nuclei were counterstained with DAPI (Beyotime, Beijing, China, C1002). Images were obtained using a confocal microscope (Olympus, Tokyo, Japan, FV1200). Primary antibodies included MVH (Abcam, Cambridge, UK, ab13840, 1:100) and CKIT (Invitrogen, California, USA, 14-1172-81, 1:100). Secondary antibodies included goat anti-rat IgG (Proteintech, Chicago, USA, SA00003-11, 1:1000, FITC labeled) and goat anti-mouse IgG (Proteintech, Chicago, USA, SA00003-12, 1:1000, TRITC labeled). The directly labeled antibody was SSEA-1 (Biotechne, Minnesota, USA, IC2155T, 1:1000). PGCs were used as a positive control, and iPSCs were employed as a negative control. Karyotype analysis A total of 1 × 10 6 iPSCs were treated with 0.25 µg/mL colchicine (TCI, Shanghai, China, C0380) and cultured in Dulbecco’s modified Eagle’s medium (DMEM) (HyClone, Utah, USA, SH30022.01B) with high glucose and 10% FBS (Gibco, New York, USA, 16000−044) for 4 h. The cells were then collected and treated with a low osmotic solution of potassium chloride (Shanghai test, Shanghai, China, 67-56-1), fixed with methanol (Shanghai test, Shanghai, China, 7447-40-7) and stained with Giemsa (Solarbio, Beijing, China, G1015) (Schmid M et al., 1989). A 100×10 oil immersion microscope (Olympus, Tokyo, Japan, BX41) was used for observation. PAS glycogen staining Cells were incubated with 4% paraformaldehyde at room temperature for 30 min and washed twice in PBS. After drying, the cells were stained with a PAS staining kit (Solarbio, Beijing, China, G1280). The samples were then treated with oxidant for 10 min and washed twice with PBS. Schiff stain solution was added to the samples for 15 min after drying. The samples were then washed twice with sulfite before washing twice with PBS and stained with hematoxylin for 2 min followed by washing twice with PBS. Images were collected using a fluorescence inverted microscope (Olympus, Tokyo, Japan, IX51). Frozen sections iPGCs, PGCs, and CEFs labeled with pKH26 cell membrane red fluorescence (Sigma, Missouri, USA, PKH26GL) were injected into 2.5-day chicken embryo blood vessels. The eggs were continuously hatched. Embedding agent for frozen sections (OCT, Cell Path, UK, 80202-0001) was added to the isolated genital ridge from the 4.5-day hatched recipient embryo. A frozen microtome (Leica, Dresden, German, CM1950) was used for sectioning (8 μm). Frozen sections were then adhered to glass slides. The migratory ability of different cells in recipient chicken embryos was identified by observing the red and green fluorescence with a fluorescence microscope (Olympus, Tokyo, Japan, IX51). Chick embryo vascular injection The 2.5-day hatched eggs (H&H 17) were collected. The blunt end of the chicken embryo was opened with a diameter hole of 1 cm after wiping the blunt ends with 75% alcohol. One microliter of cell suspension (5000 cells/μL) was injected into the blood vessel with a microinjection needle under a stereomicroscope (Olympus, Tokyo, Japan, DP72) after removing the air chamber. Then, 20 μL of penicillin (Solarbio, Beijing, China, P1400-100) was gently dripped to the opened hole. Medical paper tape was used to seal the hole with a cross method. The injected eggs were then transferred back to an incubator for continuous hatching. Statistical analysis Data from individual experiments are presented as the mean ± SEM. Differences between each group were determined to be significant using one-way ANOVA (* p < 0.05, significant; ** p < 0.01, *** p < 0.001, highly significant, the Multiple Comparisons by Tukey) or analyzed by unpaired two-tailed t -test (* p < 0.05, significant; ** p < 0.01, *** p < 0.001, highly significant). All experiments were repeated at least three times. GraphPad Prism 7.0 software was used for mapping, and flow cytometric images were analyzed by Flow Jo (Becton, Dickinson & Company). Reporting summary Further information on research design is available in the Nature Research Reporting Summary linked to this article.